Selectivity mechanism of the mechanosensitive channel MscS revealed by probing channel subconducting states The mechanosensitive channel of small conductance (MscS) has been characterized at both functional and structural levels and has an integral role in the protection of bacterial cells against hypoosmotic shock. Here we investigate the role that the cytoplasmic domain has in MscS channel function by recording wild-type and mutant MscS single-channel activity in liposome patches. We report that MscS preferentially resides in subconducting states at hyperpolarising potentials when Ca 2+ and Ba 2+ ions are the major permeant cations. In addition, our results indicate that charged residues proximal to the seven vestibular portals and their electrostatic interactions with permeating cations determine selectivity and regulate the conductance of MscS and potentially other channels belonging to the MscS subfamily. Furthermore, our findings suggest a role for mechanosensitive channels in bacterial calcium regulation, indicative of functions other than protection against osmolarity changes that these channels possibly fulfil in bacteria. Mechanosensitive channel of small conductance (MscS) was the first bacterial ion channel examined by patch clamp that was shown to respond to membrane stretch [1] . It is also the first mechanosensitive (MS) channel shown to be gated by the bilayer mechanism [2] . Since the cloning of the mscS gene [3] , MscS has emerged as an archetype of a diverse family of MS channels encompassing a number of representatives from bacteria, archaea, fungi and plants [4] , [5] . The availability of the three-dimensional (3D) MscS crystal structure [6] , [7] allows for detailed structure and function studies, and studies of bilayer effects on the gating of this channel. It functions as an emergency release valve that responds to sudden changes in environmental osmolarity by opening a large, weakly anion-selective pore of ~1-nS conductance [1] , [8] , helping to relieve excessive cellular turgor [3] . MscS forms a heptameric channel, whose 3D structure in the closed [9] , intermediate [6] , [10] and open [11] , [12] ( Fig. 1a ) conformation is available, and which has been further characterized by biochemical [13] , electrophysiological [14] , [15] , spectroscopic [11] , [16] and theoretical modelling studies [17] , [18] , [19] , [20] . 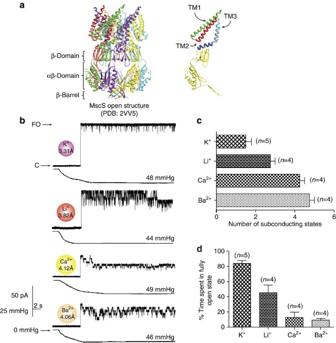Figure 1: MscS 3D structure and gating properties in the presence of monovalent and divalent cations. (a) Left panel is the structure of MscS in the open state (PDB: 2VV5) with each of the seven monomers displayed as a different colour. The right panel shows a single monomer of MscS from the open structure illustrating the TM1 (green), TM2 (red) helices and the TM3 helix which lines the pore (TM3 is split into TM3a light blue and TM3b dark blue). (b) Representative traces of MscS activity reconstituted in azolectin liposomes at +70 mV pipette potential in inside-out patches under symmetrical solutions containing: KCl 200 mM, LiCl 200 mM, BaCl2100 mM and CaCl2100 mM supplemented with HEPES 5 mM pH 7.4. The hydrated ionic radius of each permeant ion is shown for comparison. The pressure recordings applied manually are shown beneath for each trace. The pressure threshold of activation for MscS was not statistically different in these recording solutions (that is, KCl: 45.5±3.6 mm Hg, LiCl: 42.5±1.5 mm Hg, BaCl2: 48.4±5.3 mm Hg, CaCl2: 51.21±12.7 mm Hg). (c) Histograms illustrating the average number of subconducting states seen at +70 mV pipette potential during a 10 s record in symmetrical solutions as described above. Bar represent means of N numbers as stated ±s.e.m. (d) Histograms illustrating the percentage of time MscS spends in the fully open state under constant pressure application over 5 s in symmetrical solutions as described above. Bar represent means of N numbers as stated±s.e.m. C, closed; FO, fully open. Figure 1: MscS 3D structure and gating properties in the presence of monovalent and divalent cations. ( a ) Left panel is the structure of MscS in the open state (PDB: 2VV5) with each of the seven monomers displayed as a different colour. The right panel shows a single monomer of MscS from the open structure illustrating the TM1 (green), TM2 (red) helices and the TM3 helix which lines the pore (TM3 is split into TM3a light blue and TM3b dark blue). ( b ) Representative traces of MscS activity reconstituted in azolectin liposomes at +70 mV pipette potential in inside-out patches under symmetrical solutions containing: KCl 200 mM, LiCl 200 mM, BaCl 2 100 mM and CaCl 2 100 mM supplemented with HEPES 5 mM pH 7.4. The hydrated ionic radius of each permeant ion is shown for comparison. The pressure recordings applied manually are shown beneath for each trace. The pressure threshold of activation for MscS was not statistically different in these recording solutions (that is, KCl: 45.5±3.6 mm Hg, LiCl: 42.5±1.5 mm Hg, BaCl 2 : 48.4±5.3 mm Hg, CaCl 2 : 51.21±12.7 mm Hg). ( c ) Histograms illustrating the average number of subconducting states seen at +70 mV pipette potential during a 10 s record in symmetrical solutions as described above. Bar represent means of N numbers as stated ±s.e.m. ( d ) Histograms illustrating the percentage of time MscS spends in the fully open state under constant pressure application over 5 s in symmetrical solutions as described above. Bar represent means of N numbers as stated±s.e.m. C, closed; FO, fully open. Full size image The structure of the MscS monomer consists of three transmembrane helices, TM1–TM3, with the N- and C-terminal domains located on the periplasmic and cytoplasmic sides of the bacterial cell membrane, respectively. This monomer structure is based on the X-ray crystal structure of an intermediate conformation of the MscS channel from Escherichia coli [6] . According to this structure, the pore of the MscS channel is formed by seven TM3 helices. Initially, its unitary conductance of ~1 nS, non-saturability in high salt and weak anion selectivity suggested a water-filled open channel pore of ~16 Å in diameter [21] , which was later confirmed by structural studies [22] . TM1 and TM2 helices function as the sensors for membrane tension and are involved in channel voltage sensitivity [6] , [23] , [24] . The role of the MscS cytoplasmic vestibular domain in channel function is less well understood. The current view is that the chamber is a dynamic structure that undergoes significant conformational change upon channel gating [25] , [26] . During gating the cytoplasmic vestibulum passively follows the movement of the ‘hairpin’ formed by the transmembrane TM1 and TM2 helices [6] , [27] , [28] as well as the expansion of the aqueous pore, lined by the TM3 helices [15] , [26] . The cytoplasmic domain is also considered to have a role in the adaptation and inactivation of the channel [25] , [26] , [29] and has been suggested to serve as a sensor for cytoplasmic crowding [19] , [30] . Furthermore, it has been proposed that the MscS cytoplasmic vestibulum may have the role of an ion-selectivity filter in this channel [6] , [20] , [31] , [32] . Since the first report demonstrating a relatively weak level of anion selectivity ( P Cl / P K =2.7) ( Supplementary Table S1 ) [1] , a number of studies have reported similar MscS preference for anions over cations. To account for this observation, the seven vestibular portals in the MscS cytoplasmic chamber have been suggested to act as selectivity filters [6] , [19] , [20] . The notion that MscS ion selectivity may be mediated through creation of ‘ion clouds’ around the seven portals is supported by a study showing that pore mutations of the MscS channel affected channel desensitization but not its ionic preference [31] . In this study, we have addressed this hypothesis by examining MscS conductance, ion selectivity and gating properties in solutions containing different mono- and divalent cations. We compared the selectivity of several members of the MscS-like channel subfamily, whose ion-conducting properties were previously investigated and reported [32] , [33] , [34] , [35] , [36] , [37] , [38] , using them as natural variations of the vestibular primary structure reflected by their ion selectivity. Furthermore, we also mutagenized two carefully chosen charged residues within the cytoplasmic chamber of MscS of E. coli. Our choice was based on detailed analysis of the possible effects of different mutations on the electronegative area within the vestibulum of MscS (see Results). Together, these data provide strong evidence for the role of the C-terminal domain as a selectivity filter in MscS-like channels. Our study indicates further that divalent cations have an important role for MscS’ conductive properties by favouring the channel gating at subconducting levels. Furthermore, and perhaps most interestingly of all, we show that on opening, MS channels can become not only a passageway for osmolyte exit, but also a conduit for the entry of ions including Ca 2+ . Our results have important implications for the physiology of bacterial cells. Modulation of MscS gating by monovalent and divalent cations Single-channel recordings obtained from MscS in a recording solution containing KCl at positive pipette potentials ≥+70 mV over a 5-s period revealed that the channels spent on an average ≥80% of the time in the fully open state. The tendency of MscS to gate at subconducting levels was more pronounced in the recording solution containing LiCl and significantly pronounced in CaCl 2 and BaCl 2 ( Fig. 1b and c ). MscS only spent <20% and <12% of the time, respectively, in the fully open state in the presence of CaCl 2 and BaCl 2 ( Fig. 1d ). For the rest of the 5-s period, the channels were gating exclusively at subconducting levels in the presence of these cations ( Figs 2 and 3 ). Whereas forays into substates at pipette potentials ≥+70 mV in KCl and LiCl were short-lived, once subconducting states were entered in the recording solutions containing CaCl 2 and BaCl 2 , the channels did not revert to the fully open state ( Figs 1b , 2 and 3 ). In addition, the number of subconducting states observed at the same pipette potential in the presence of monovalent cations (K + and Li + ) was markedly lower than that seen in the presence of divalent cations (Ca 2+ and Ba 2+ ) ( Fig. 1c ). As discussed further in the text, it appears that the tendency for the channel to reside in subconducting states correlates strongly with the hydrated ionic radii of the major permeant cation ( Fig. 1 ). 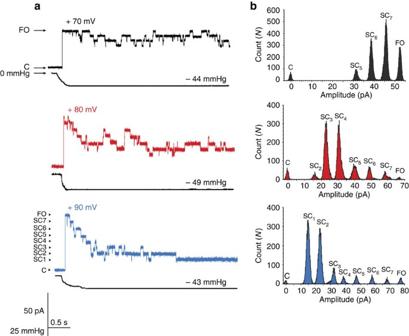Figure 2: Subconducting states in MscS in the presence of Ba2+. (a) Raw records of MscS activity reconstituted in azolectin liposomes at +70, 80 and 90 mV pipette potential in inside-out patches under symmetrical conditions (BaCl2100 mM, HEPES 5 mM, pH 7.4). Numerous long-lived subconducting states were observed with the number increasing with voltage. Pressure traces of manually applied negative pressure (suction), using a syringe, are shown beneath each recording. (b) Distribution of current histograms from raw records depicted in (a) illustrating the rise in the number of subconducting states with increasing pipette voltage to a maximum of 8 conducting states. C, closed; FO, fully open; SC, subconducting state. Figure 2: Subconducting states in MscS in the presence of Ba 2+ . ( a ) Raw records of MscS activity reconstituted in azolectin liposomes at +70, 80 and 90 mV pipette potential in inside-out patches under symmetrical conditions (BaCl 2 100 mM, HEPES 5 mM, pH 7.4). Numerous long-lived subconducting states were observed with the number increasing with voltage. Pressure traces of manually applied negative pressure (suction), using a syringe, are shown beneath each recording. ( b ) Distribution of current histograms from raw records depicted in ( a ) illustrating the rise in the number of subconducting states with increasing pipette voltage to a maximum of 8 conducting states. C, closed; FO, fully open; SC, subconducting state. 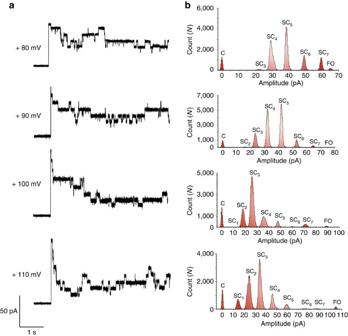Figure 3: MscS subconducting states in the presence of Ca2+. (a) Raw records of MscS activity reconstituted in azolectin liposomes at +80, 90, 100 and 110 mV pipette potential in inside-out patches under symmetrical conditions (CaCl2100 mM, HEPES 5 mM, pH 7.4). Similarly to the activity observed in BaCl2numerous long-lived subconducting states are present with the number increasing with voltage up to a maximum of eight conducting states. Applied pressure was manually applied and was comparable to that shown inFigs 1and2(40–60 mm Hg). (b) Distribution of current histograms from raw records depicted in (a) illustrating the rise in the number of subconducting state with increasing pipette voltage to a maximum of 8 conducting states as seen with BaCl2. C, closed; FO, fully open; SC, subconducting state. Full size image Figure 3: MscS subconducting states in the presence of Ca 2+ . ( a ) Raw records of MscS activity reconstituted in azolectin liposomes at +80, 90, 100 and 110 mV pipette potential in inside-out patches under symmetrical conditions (CaCl 2 100 mM, HEPES 5 mM, pH 7.4). Similarly to the activity observed in BaCl 2 numerous long-lived subconducting states are present with the number increasing with voltage up to a maximum of eight conducting states. Applied pressure was manually applied and was comparable to that shown in Figs 1 and 2 (40–60 mm Hg). ( b ) Distribution of current histograms from raw records depicted in ( a ) illustrating the rise in the number of subconducting state with increasing pipette voltage to a maximum of 8 conducting states as seen with BaCl 2 . C, closed; FO, fully open; SC, subconducting state. Full size image Ba 2+ and Ca 2+ conductance In the presence of symmetrical 100 mM BaCl 2 , the unitary conductance of the fully open MscS channel at positive and negative pipette potentials was g + =555±24 pS ( n =12) and g − =354±17 pS ( n =12), respectively ( Figs 2a and 4a ). Hence, in BaCl 2 the conductance at positive pipette potentials was 1.57-times higher than at negative pipette potentials. Importantly, in our experiments, irrespective of the ion species present, the channels always rectified in the same direction because the reconstituted MscS channels in all our experiments were oriented the same way, that is, the right-side-out orientation. As shown in Supplementary Fig. S1 , the channels are oriented the same way as in the native membrane of inside-out excised patches of giant bacterial spheroplasts, meaning that the periplasmic (extracellular) side of MscS was facing the interior of the patch pipettes, whereas the cytoplasmic C-terminal domain was facing the bath solution. This result is in agreement with previously published MscS studies reporting a ‘non-random orientation’ of channels in liposome membranes [21] . Our evidence here for the uniform right-side-out orientation of MscS is based on the fact that trifluoroethanol (TFE) application to the bath (cytoplasmic side) increased MscS inactivation, whereas TFE applied from the pipette did not have any effect, as previously reported [39] ( Supplementary Fig. S1 ). This result mirrors what is seen in MscL channels, which also orientate themselves right-side out upon reconstitution into liposomes [40] . 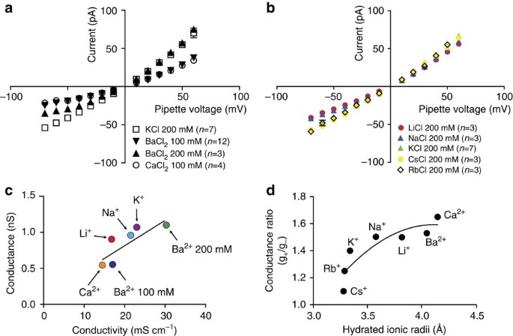Figure 4: MscS rectification in the presence of different monovalent and divalent cations. (a) Current-voltage plot for MscS reconstituted in azolectin liposomes in the presence of symmetrical KCl 200 mM, CaCl2100 mM, BaCl2100 mM and BaCl2200 mM, HEPES 5 mM, pH 7.4. Current-voltage plot generated from amplitudes of fully open channels. There is a larger degree of rectification at negative pipette potentials in the presence of Ba2+and Ca2+than when K+is the major permeant cation. Applied pressures were between 40 and 60 mm Hg. (b) Current-voltage plots for MscS in the presence of equimolar alkali metal chlorides. An increase in rectification is seen as the hydrated ionic radius of the major permeant cation is increased. Current-voltage plot generated from amplitudes of fully open channels. (c) Unitary conductance of MscS (fully open state) at positive pipette potentials plotted against corresponding measured bulk conductivities of recording solutions fitted with a linear regression line (R2=0.644). (d) Illustration of how MscS rectification (plotted as ratio of conductance at positive potentials against negative potentials of fully open channels) changes with the hydrated ionic radii of the major permeant cation. Figure 4: MscS rectification in the presence of different monovalent and divalent cations. ( a ) Current-voltage plot for MscS reconstituted in azolectin liposomes in the presence of symmetrical KCl 200 mM, CaCl 2 100 mM, BaCl 2 100 mM and BaCl 2 200 mM, HEPES 5 mM, pH 7.4. Current-voltage plot generated from amplitudes of fully open channels. There is a larger degree of rectification at negative pipette potentials in the presence of Ba 2+ and Ca 2+ than when K + is the major permeant cation. Applied pressures were between 40 and 60 mm Hg. ( b ) Current-voltage plots for MscS in the presence of equimolar alkali metal chlorides. An increase in rectification is seen as the hydrated ionic radius of the major permeant cation is increased. Current-voltage plot generated from amplitudes of fully open channels. ( c ) Unitary conductance of MscS (fully open state) at positive pipette potentials plotted against corresponding measured bulk conductivities of recording solutions fitted with a linear regression line ( R 2 =0.644). ( d ) Illustration of how MscS rectification (plotted as ratio of conductance at positive potentials against negative potentials of fully open channels) changes with the hydrated ionic radii of the major permeant cation. Full size image As mentioned above, in the presence of BaCl 2 multiple long-lived subconducting states were observed above +70 mV pipette potential ( Figs 1b and 2 ). The number of subconducting states increased as pipette potential increased with a maximum of eight conducting states being observed at +90 mV ( Fig. 2a ). No additional conducting states were observed up to a maximum pipette potential of +140 mV applied to membrane patches in this study. These substates were examined at positive pipette potentials (corresponding to negative membrane potentials in our recordings) because the physiological membrane potential of E. coli is estimated to be around −150 mV (ref. 41 ), and substates at positive pipette potentials are easier to distinguish than at negative potentials. Furthermore, there are very few reports of MscS subconducting behaviour at positive pipette potentials. Interestingly, the channels always entered the fully open state before entering any substates, there being no example of a closed state-to-subconducting state transition identified during this study. Furthermore, the time the channel spent in the fully open state decreased with increasing pipette voltage. Once the pipette potential exceeded +90 mV, on occasion, the channel continued gating at the lowest subconducting states (SC1–3) after constant negative pressure (between 40–60 mm Hg) was removed. The magnitude of applied pressure did not correlate with this phenomenon, that is, as applied pressure increased the likelihood for gating after pressure removal did not increase. Similar behaviour was seen in CaCl 2 ( Fig. 3 , Supplementary Table S2 ), although slight differences were observed. In the presence of symmetrical BaCl 2 , the channel favoured occupancy of the lowest substates (SC1 and SC2; Fig. 2 ), whereas in symmetrical CaCl 2 the channel seemed to favour other substates (SC3 and SC4; Fig. 3 ). The unitary conductance of the fully open MscS channel at positive pipette potentials and negative pipette potentials was g + =547±35 pS and g − =337±24 pS in 100 mM CaCl 2 , respectively ( n =5) ( Fig. 4a ). The conductance at positive pipette potentials is therefore 1.62-times higher than at negative pipette potentials ( Fig. 4a ). Consequently, it appears that MscS conductance rectifies in the same way irrespectively of the ion species carrying the current [1] , [8] , [21] . However, as discussed further, the extent to which MscS conductance rectifies is dependent on the permeant ions ( Fig. 4b ). The structural basis of MscS subconducting states As previously reported, the MscS vestibular portals have no real distinguishing features [19] . There are numerous polar and apolar residues surrounding the ~13-Å diameter perforations [10] . One point to note, however, is the highly electronegative region inside the vestibule proximal to each portal centred around two glutamic acid residues, E187 and E227 (ref. 19 ). We hypothesized that the eight conducting states observed arose from intermittent occlusion of the seven lateral vestibular portals through electrostatic interactions with permeating cations. In order to further explore this idea, we estimated the size of the pore corresponding to the lowest MscS subconductance state (SC1) and compared it to the size of the vestibular portals and the central ‘pore’ coaxial with the channel pore determined from the MscS 3D structure [6] (PDB accession code 2VV5 ). This calculation is shown in the Methods section. It is important to note, however, that some simulation studies indicate ionic movement through the ‘pore’ aligned coaxially to the transmembrane pore is unlikely [10] . Nevertheless, given that the chimera composed of the transmembrane portion of Thermoanaerobacter tengcongensis MscS and β-barrel of E. coli MscS was still active [32] , we cannot completely exclude the possibility that the β-barrel pore of MscS has a role in ion permeation with ions moving through the pore at the rate corresponding to the smallest observed substate SC1 in this study. MscS also displays characteristic voltage dependent-inactivation. In this study, although no quantitative analysis was performed, we did not encounter any noticeable MscS inactivation (without TFE present). There are two possible reasons for this; firstly, MscS inactivation is much slower at hyperpolarising potentials (positive pipette potentials), and secondly, it is blunted in azolectin liposomes possibly due to lipid composition [21] , [29] . Sukharev and coworkers [29] suggest that MscS proceeds through substates into the inactivated state. From this we may extrapolate that the presence of divalent cations such as Ba 2+ and Ca 2+ may influence these transitions resulting in a higher occupancy of substates. This could be via interactions with the cytoplasmic domain or through allosteric modulation of the pore helices. The effect of hydrated ionic radii on MscS rectification In the presence of 100 mM CaCl 2 and BaCl 2 , there was greater rectification at negative pipette potentials than when monovalent cations were the major permeant ions ( Fig. 4a ). Figure 4a shows a comparison between 100 mM BaCl 2 , 100 mM CaCl 2 , 200 mM BaCl 2 and 200 mM KCl. The unitary conductance of the fully open MscS channel for each ionic species at positive potentials, was g + =555±24 pS ( n =12), g + =547±35 pS ( n =5), 1110±72 pS ( n =3) and 1078±30 pS ( n =7), respectively ( Fig. 4a ). The measured bulk conductivities of these solutions were 17 mS cm −1 , 15 mS cm −1 , 23 mS cm −1 and 30 mS cm −1 , respectively, which partly explains these conductance differences ( Fig. 4c ). This effect of bulk conductivity against MscS conductance (fully open state) at positive potentials is illustrated in Fig. 4c . Another factor, which can also explain and contribute to these conductance differences, is stronger MscS selectivity for anions in the presence of divalent cations, which is probably due to stronger binding of Ba 2+ and Ca 2+ to the electronegative surface in the MscS vestibulum. This notion is supported by the fact that the current amplitude is bigger in both E187R and E227A mutants exhibiting weaker anion selectivity than the wild-type MscS ( Fig. 5 ; Supplementary Table S3 and Supplementary Fig. S2 ) (see further in text). The unitary conductance of the fully open MscS channel at negative pipette potentials in 100 mM BaCl 2 , 100 mM CaCl 2 200 mM BaCl 2 and 200 mM KCl was g − =354±17 pS ( n =12), g − =337±24 pS ( n =5), 634±32 pS ( n =3) and 804±26 pS ( n =7), respectively ( Fig. 4a ). The rectification ratios g + / g − were therefore 1.57, 1.62, 1.75 and 1.35, respectively. 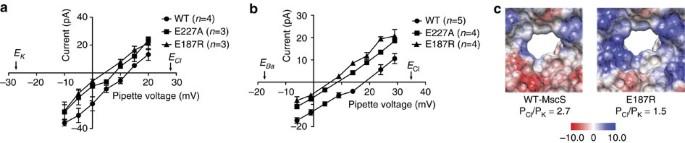Figure 5: MscS mutants E187R and E227A exhibit weaker anion selectivity than wild-type (WT)-MscS. (a) Current-voltage plots for WT-MscS, E187R and E227A mutant channels reconstituted in azolectin liposomes in asymmetric solutions (600 mM KCl pipette/200 mM KCl bath, HEPES 5 mM pH 7.4). The mutants exhibit reversal potentials that are further fromEClthus demonstrating lower anion selectivity than the WT channel. (calculatedErevpipette;EK=−28 mV andECl=+28 mV). (b) Current-voltage plots for WT-MscS, E187R and E227A mutant channels reconstituted in azolectin liposomes in asymmetric solutions (200 mM BaCl2pipette/50 mM BaCl2bath, HEPES 5 mM pH 7.4). The mutants exhibit reversal potentials that are further fromEClthus demonstrating lower anion selectivity than the WT channel. (calculatedErevpipette;EBa=−18 mV andECl=+35 mV). (c) Coulombic charge maps of WT-MscS and E187R mutant vestibular portals as viewed from inside the cytoplasmic domain (kcal mol−1eat 298 K) (also see SupplementaryFig. S2). Figure 5: MscS mutants E187R and E227A exhibit weaker anion selectivity than wild-type (WT)-MscS. ( a ) Current-voltage plots for WT-MscS, E187R and E227A mutant channels reconstituted in azolectin liposomes in asymmetric solutions (600 mM KCl pipette/200 mM KCl bath, HEPES 5 mM pH 7.4). The mutants exhibit reversal potentials that are further from E Cl thus demonstrating lower anion selectivity than the WT channel. (calculated E rev pipette; E K =−28 mV and E Cl =+28 mV). ( b ) Current-voltage plots for WT-MscS, E187R and E227A mutant channels reconstituted in azolectin liposomes in asymmetric solutions (200 mM BaCl 2 pipette/50 mM BaCl 2 bath, HEPES 5 mM pH 7.4). The mutants exhibit reversal potentials that are further from E Cl thus demonstrating lower anion selectivity than the WT channel. (calculated E rev pipette; E Ba =−18 mV and E Cl =+35 mV). ( c ) Coulombic charge maps of WT-MscS and E187R mutant vestibular portals as viewed from inside the cytoplasmic domain (kcal mol −1 e at 298 K) (also see Supplementary Fig. S2 ). Full size image Subsequently, equimolar alkali metal chlorides were tested in turn to see whether any differences in rectification could be identified for these cations ( Fig. 4b ). More rectification was seen in the presence of NaCl and LiCl ( g + / g − ratio: 1.51 and 1.50, respectively) with the least rectification seen with CsCl ( g + / g − ratio: 1.15). After testing all the alkali cations, the results indicated that the larger the hydrated ionic radius of the major permeant cation the greater the degree of g + /g − rectification ( Fig. 4d ). Hence, it seems the energy of interaction between the electronegative MscS site and a cation is dominated by the hydration energy of interaction between the site and a permeant cation. The ion-exchange equilibrium at the particular MscS site is best described by the Eisenman sequence I, which is well approximated by the sequence Cs + >Rb + >K + >Na + ~Li + indicated in Fig. 4d . We hypothesize that a weak field strength resulting from the electronegative region inside the vestibule, possibly centred around positions E187 and E227, contributes to the observed MscS-rectifying conductive properties. We further compared the conductance ratios ( g + / g − ), in the presence of symmetrical 100 mM CaCl 2 and BaCl 2 , and as shown above, we obtained g + / g − ratio of 1.62 and 1.57, respectively ( Fig. 4d ), similar to the results obtained with Li + and Na + ions. We interpret this result as an indication that steric effects resulting from the obstruction of the passage of ions at the cytoplasmic entrance of the channel may be the cause of rectification, as previously suggested [19] . According to the Eisenman model of ion selectivity, Eisenman sequence I would imply that the energy of interaction between the site and the permeant cation is small, meaning that ion exchange is dictated by the dehydration energy, which among alkali metal ions is lowest for Cs + (−71 kcal mol −1 ), and highest for Li + (−131 kcal mol −1 ). While we propose this site to be important for rectification, we cannot rule out other contributing factors likely situated within the transmembrane domain. E187R and E227A exhibit weaker anion selectivity If cations were to interact with the electronegative region at E187 and E227 sites inside the cytoplasmic vestibule proximal to the lateral portals, then this would effectively result in screening of the negative charges, thus, making anion transport more favourable in the presence of larger divalent cations. This idea of anion selectivity was first put forward by Franciolini and Nonner [42] ( Fig. 7 ). This is indeed what is seen with the P Cl / P Ba being 3.9, P Cl / P Ca being 3.7 and the P Cl / P K being 2.7 ( Fig. 5 and Supplementary Table S3 ). To test the possibility that E187 and E227 are important structural determinants of the observed MscS substates, the following mutants were created: E187R and E227A. Although these mutants showed no noticeable differences in the size of subconducting states (see Supplementary Fig. S2 ), they did exhibit modified anion selectivity ( Fig. 5 and Supplementary Table S3 ). Reports of MscS selectivity vary as shown in Supplementary Table S1 ( P Cl / P K ~1.2–3). Previous work has also demonstrated that this small anion selectivity is not a functional property of the pore-lining TM3 helix or β-barrel, as mutations in these regions have no impact on ion selectivity [31] . Indeed inspection of six electrophysiologically characterized MscS homologues with differing levels of anion and cation selectivity reveals that the putative pore-lining residues are mainly hydrophobic, and illustrate no major descriptors for ionic selectivity ( Supplementary Fig. S3 ). 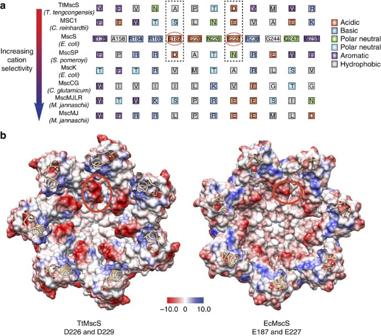Figure 6: Comparison of cytoplasmic domains of MscS subfamily. (a) Multiple sequence alignment of vestibular portal residues of electrophysiologically characterized MscS homologues with differing selectivity. The residues circled are those mutated in this study. (b) Coulombic charge distribution of a transverse section as viewed from the extracellular side ofE. coliMscS (PDB: 2VV5; right panel) andThermoanaerobacter tengcongensisMscS (PDB: 3T9N; left panel) (kcal mol−1eat 298 K). A stronger region of electronegativity in a similar location to that seen inE. coliMscS is seen inT. tengcongensisMscS. This supports the idea that MscS selectivity is brought about via ion binding/trapping in the cytoplasmic domain. Figure 6: Comparison of cytoplasmic domains of MscS subfamily. ( a ) Multiple sequence alignment of vestibular portal residues of electrophysiologically characterized MscS homologues with differing selectivity. The residues circled are those mutated in this study. ( b ) Coulombic charge distribution of a transverse section as viewed from the extracellular side of E. coli MscS (PDB: 2VV5; right panel) and Thermoanaerobacter tengcongensis MscS (PDB: 3T9N; left panel) (kcal mol −1 e at 298 K). A stronger region of electronegativity in a similar location to that seen in E. coli MscS is seen in T. tengcongensis MscS. This supports the idea that MscS selectivity is brought about via ion binding/trapping in the cytoplasmic domain. Full size image We report here that the reversal potentials of E187R and E227A in both BaCl 2 and KCl approached that of the equilibrium potentials of Ba 2+ and K + , respectively, indicating a lower level of anion selectivity compared to WT-MscS. The Coulombic charge map generated for the E187R mutant illustrates that the highly electronegative region seen in WT-MscS is likely to be completely abolished in the mutant ( Fig. 5c and Supplementary Fig. S2 ). Thus E187R and E227A are the first MscS mutant channels that exhibit modified anion selectivity. The reason for choosing these mutants was first, that they formed the centre of the electronegative region identified inside the cytoplasmic domain. Secondly, that multiple sequence alignment shows that MscK has an alanine at the corresponding position to E227 in MscS, in addition to lacking an acidic residue at the equivalent position of E187, and MscK exhibits almost no anion selectivity ( Fig. 6a ) [33] . As a result, E187 was mutated to an arginine to have the largest effect on this electronegative region and E227 was mutated to alanine to mimic MscK. Six other electrophysiologically characterized MscS homologues were also studied: MscCG from Corynebacterium glutamicum [35] , Thermoanaerobacter tengcongensis MscS [32] , MSC1 from Chlamydomonas reinharditii [37] , MscSP from Silicibacter pomeroyi [38] , and MscMJ and MscMJLR from Methanococcus jannaschii [34] . All MscS homologues have large putative cytoplasmic domains [32] ( Supplementary Fig. S4 ). Multiple alignments of 12 residues, which form or lie within close proximity to the cytoplasmic portals in MscS with the seven electrophysiologically characterized homologues, are shown in Fig. 6a . An acidic residue at position 187 in MscS is not conserved in the anion-selective channel MSC1 but the acidic residue at position 227 is conserved, the opposite being true of the anion-selective MscSP (ref. 38 ). Notably, MSC1 displays markedly more anion selectivity than MscS and while no corresponding acidic residue is found at E187, there is an acidic residue in MSC1 that aligns at position 247 in MscS. An acidic residue at this position could contribute towards anion selectivity in MSC1 through cation binding/trapping in a similar fashion hypothesized for MscS. In addition, recent evaluation of an MscS homologue from T. tengcongensis convincingly implicates the role of the β-barrel in the selectivity of this channel. However, the residual strong anion selectivity of T. tengcongensis MscS mutant E278A could be explained by a similar paradigm to that suggested in this study. As shown in Fig. 6b , T. tengcongensis MscS also exhibits a highly electronegative region in the cytoplasmic domain. So, while the β-barrel seems to be important for the anion selectivity in T. tengcongensis MscS, the cytoplasmic vestibule may also have a role similar to that shown in E. coli MscS ( Fig. 5 ) [32] . As previously mentioned, this selectivity paradigm resembles the anion selectivity mechanism initially proposed by Franciolini and Nonner [42] ( Fig. 7 ). 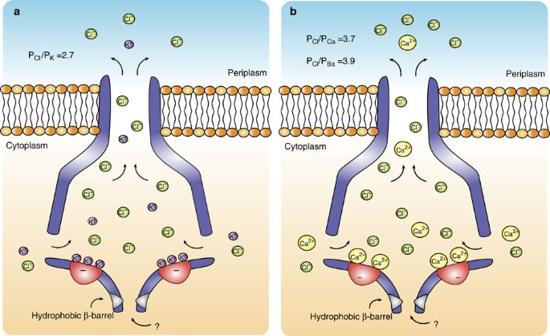Figure 7: Graphic illustration of proposed MscS selectivity mechanism. (a) Cations such as K+bind to the electronegative region comprised of residues including E187 and E227 (shown in red). The binding/trapping of cations in these areas or ‘ion clouds’ makes anion transport more favourable and results in the larger cation transit time calculated in molecular dynamic simulations20. (b) As the size of the co-permeant cation gets larger (depicted as Ca2+) in turn there is a larger effect on both cation and anion transport resulting in higher anion selectivity. This explanation does not preclude cation transport totally and the distance of this region from the lateral vestibular portals probably accounts for the weak level of anion selectivity exhibited. Figure 7: Graphic illustration of proposed MscS selectivity mechanism. ( a ) Cations such as K + bind to the electronegative region comprised of residues including E187 and E227 (shown in red). The binding/trapping of cations in these areas or ‘ion clouds’ makes anion transport more favourable and results in the larger cation transit time calculated in molecular dynamic simulations [20] . ( b ) As the size of the co-permeant cation gets larger (depicted as Ca 2+ ) in turn there is a larger effect on both cation and anion transport resulting in higher anion selectivity. This explanation does not preclude cation transport totally and the distance of this region from the lateral vestibular portals probably accounts for the weak level of anion selectivity exhibited. Full size image MscS ion selectivity and bacterial physiology Measurement of free Ca 2+ in E. coli using recombinant aequorin has shown that, like eukaryotic cells, bacteria maintain a low cytosolic free Ca 2+ in the sub-micromolar to micromolar range in the presence of mM Ca 2+ extracellularly [43] , [44] , [45] . Furthermore, the Donnan potential across the outer membrane means that free Ca 2+ in the periplasmic space may be higher than in the external medium [46] . Microarray analysis showed that a rise in cytosolic free Ca 2+ regulated at least 90 genes [47] . Perhaps unsurprisingly, single knockouts (KOs) of the mechanosensitive channels MscL and MscS exhibited no differences in Ca 2+ influx or efflux compared with the wild-type [47] . However, the results reported here illustrate that MscS, as well as MscL and MscK, are freely permeable to divalent ions such as Ca 2+ . Therefore, a key question is—under physiological conditions in live cells, can mechanosensitive channels let Ca 2+ into the cell? Given the toxicity of excessive calcium concentration for living cells, we suggest that the regulation of the MscS selectivity, rectifying properties and subconducting states by divalent ions Ba 2+ and Ca 2+ reported here may represent another mechanism of bacterial calcium regulation, in particular under life-threatening conditions. Challenged by a hypoosmotic shock, bacteria are forced to open their MS channels [3] . The large pores of MscS and other MS channels become then not only a conduit for osmolytes outward of the cell relieving excessive cellular turgor but also a pathway for extracellular ions including Ca 2+ to enter the intracellular space, which in turn could cause depolarization of the bacterial cell membrane. In order to test this hypothesis, we utilised the calcium-activated photoprotein aequorin. We found that a hypoosmotic shock equivalent to ~350 mOsm resulted in a large Ca 2+ transient in WT FRAG-1 E. coli cells (9.39 μM±1.12 μM ( n =3)). This Ca 2+ rise was significantly blunted in the triple KO MJF465 ( mscL − , mscS − and mscK − ) E. coli strain (4.65±0.11 μM ( n =3)) ( Fig. 8 ). This supports the notion that MS channels may, on opening, become gateways into the cell for external ions such as Ca 2+ . The rise in cytosolic free Ca 2+ in the MJF465 strain may be mediated by Ca 2+ influx via one or all of the other four MS channels expressed in this KO (gene products of ybdG , ybiO , ynaI and yjeP ) [48] . An important point to note is that with a hypoosmotic shock of this magnitude, there is significant MscL and MscS activity in FRAG-1 but it is not large enough, even for the MJF465 strain, to cause significant cell lysis [3] . Furthermore, while microarray analysis has shown that expression of MS channels is not regulated by Ca 2+ , the stress sigma factor, RpoS, which has been shown to modulate MS channel expression, is susceptible to changes in Ca 2+ (refs 47 , 49 ). Hence, this Ca 2+ current may be a physiological signal in vivo regulating MS channel expression. 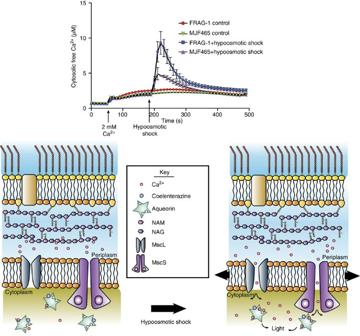Figure 8: Ca2+influx via MS channelsin vivoshown using aequorin chemiluminescence. The upper panel illustrates how a hypoosmotic shock of ~350 mOsm affects cytosolic free Ca2+in FRAG-1 (WT) and MJF465 (triple KOmscL−,mscS−andmscK−)E. colicells. The illustration below depicts how this Ca2+transient may arise. This influx of Ca2+is made possible by the large electrochemical gradient driving Ca2+entry; namely a concentration gradient of mM to low μM and a membrane potential of approximately −150 mV (ref.41). NAG,N-acetylglucosamine; NAM,N-acetylmuramic acid. Figure 8: Ca 2+ influx via MS channels in vivo shown using aequorin chemiluminescence. The upper panel illustrates how a hypoosmotic shock of ~350 mOsm affects cytosolic free Ca 2+ in FRAG-1 ( WT ) and MJF465 (triple KO mscL − , mscS − and mscK − ) E. coli cells. The illustration below depicts how this Ca 2+ transient may arise. This influx of Ca 2+ is made possible by the large electrochemical gradient driving Ca 2+ entry; namely a concentration gradient of mM to low μM and a membrane potential of approximately −150 mV (ref. 41 ). NAG, N -acetylglucosamine; NAM, N -acetylmuramic acid. Full size image Ion selectivity of MscS and its homologues described in this study differs from the ion selectivity of voltage-gated K + , Na + , Ca 2+ or Cl − channels, as it is not defined by residues within the pore of the channel but originates from the charge distribution within its cytoplasmic vestibular domain. By testing permeation of major monovalent and divalent cations in the wild-type and two vestibular MscS mutants, we were able to demonstrate that the cytoplasmic chamber does not only determine the ion selectivity of MscS, and potentially other MscS-like channels, but may also control their rectifying properties. This study also shows that Ca 2+ and Ba 2+ reduce MscS conductance at hyperpolarizing membrane voltages (corresponding to positive pipette voltages in our experiments), and causes the channel to gate frequently at subconducting levels. In addition to this MS channels, such as MscS, may also act as gateways into the cell for external Ca 2+ ions. We propose that subsequent interactions with acidic residues within the cytoplasmic vestibulum help to restrict an excessive rise of intracellular calcium, which has been implicated in a number of bacterial cell functions including chemotaxis [50] . In conclusion, our findings have implications for bacterial cell physiology with regards to the regulation of intracellular calcium, in particular in cells during starvation or in those exposed to life-threatening hypoosmotic conditions. Materials All reagents unless stated otherwise were analytical grade from Sigma. Bioinformatic methods All bioinformatic programs used herein are available online. Multiple sequence alignments were obtained using CLUSTAL W. The aligned sequences were obtained from GenBank. Pair-wise sequence alignments used to generate sequence identity and similarity were carried out using EMBOSS Needle, Needleman–Wunsch alignment; EMBL-EBI. Hydropathy plots were created and mutant sequencing carried out using the DNASTAR lasergene suite. Generation of MscS mutants and protein purification Single-residue mutants of MscS housed within a pQE-70 vector flanked by a Hin dIII restriction site were achieved using a Quick change II (Stratagene, La Jolla, CA, USA) site-directed mutagenesis kit in conjunction with the associated Quick change II protocol. The primers used to generate these mutants are shown in Supplementary Table S4 . Sequencing of the resulting mutants was carried out by The Sequencing Service (Garvan Institute, Sydney, New South Wales, Australia). Full-length wild-type MscS and mutant proteins were purified as previously reported using a 6 × -His-tag [51] . Liposome preparation and electrophysiology Liposomes were formed by the dehydration–rehydration method, as previously described [52] , [53] . An aliquot of the liposome preparation (1 μl) was then added to the recording chamber. The resulting unilamellar blisters that formed on the bottom of the recording chamber were used to patch channels in the excised inside-out configuration at room temperature. Borosilicate glass microelectrodes (Drummond Scientific Co., Broomall, PA, USA) were formed using a Flaming/Brown pipette puller (P-87, Sutter Instruments Co., Novato, CA, USA). The resulting microelectrodes had resistances ranging from 2–5 MΩ. Ion channel activity subsequent to negative pressure application monitored via a piezoelectric pressure transducer (Omega Engineering, Stamford, CT, USA) was recorded using an Axon 1D patch-clamp amplifier (Axon Instruments, Forster City, CA, USA) at a sampling rate of 10 kHz and filtered at 5 kHz. Accrued single-channel data were analysed using pCLAMP10 software (Axon Instruments, Forster City, CA, USA). All monovalent ionic solutions contained 40 mM MgCl 2 and 5 mM HEPES (pH 7.4 adjusted with NaOH). All divalent ionic solutions contained 5 mM HEPES (pH 7.4 adjusted with NaOH). Relative permeabilities were calculated using the following versions of the Goldman–Hodgkin–Katz equation, where X is a monovalent cation and Y is a divalent cation: Junction potentials were calculated using JPCalc [54] and the resulting reversal potentials were adjusted accordingly. Pore diameter of the lowest subconducting state If the hypothesis regarding vestibular portal occlusion were correct then the lowest subconducting state would be a result of ion permeation via the pore aligned coaxially to the transmembrane pore alone. Permeation via this portal is not confirmed by simulation studies [5] ; however, data from chimeras of E. coli MscS and T. tengcongensis MscS imply that ion permeation via this pathway may in fact be possible [6] . In order to estimate whether the smallest subconducting state (SC1) was indeed due to permeation via the pore aligned coaxially with the transmembrane pore, a modified Hille’s equation was utilized: where ρ is the measured bulk resistivity of the solutions, which were 0.58 and 0.66 Ω cm −1 for BaCl 2 and CaCl 2 , respectively. The conductance g in BaCl 2 and CaCl 2 was estimated from the slope of an I–V plot constructed from current amplitudes of the smallest subconducting states at four potentials (242±63 pS and 250±83 pS, respectively). In this case, we estimated l from the bilayer thickness and pore length (35 or 80 Å) (ref. 6 ), which resulted in an estimated d pore in CaCl 2 and BaCl 2 to be in the rage of 5–9 Å. While the diameter of the vestibular portals is ~13 Å, the diameter of the pore aligned coaxially with the transmembrane pore is ~8 Å. Consequently, the results indicate that the lowest subconducting state may originate from permeation via the pore aligned coaxially with the membrane pore. From this we can suggest that the other subconducting states may arise as a result of the occlusion of vestibular portals. Molecular modelling The E. coli MscS crystal structure (PDB: 2VV5) was viewed in Chimera UCSF 1.6 and used to generate Coulombic charge maps at pH 7.4. Single-residue mutagenesis was also performed in Chimera UCSF 1.6 and corresponding Coulombic charge maps were generated in an identical manner. Reconstitution of active aequorin Wild-type FRAG-1 (F-, lacZ82 (Am), λ-, rha-4 , thi-1 and gal-33 ) and MJF465 (FRAG-1, ΔkefA::kan, ΔmscL::cm, ΔyggB) E. coli strains were transformed with a plasmid (pMMB66EH Amp R ) encoding for apoaequorin using heat shock. Both strains were grown to exponential phase (OD 600 : ~0.3) in LB media (1% tryptone, 0.5% yeast extract and 0.5% NaCl, pH 7.2), then grown for 2 h in the presence of 0.1 mM isopropyl β- D -thiogalactoside to induce apoaequorin expression. Subsequently, cells were incubated in the dark in the presence of 5 μM coelenterazine in order to reconstitute active aequorin. Chemiluminescence measurements and cytosolic free Ca 2+ Light emission was measured using a home-built chemiluminometer linked to a computer with results being recorded as counts per 10 s over a 5-min period and converted to free Ca 2+ using an equation from a standard curve as previously described [44] , [45] . Owing to the use of rate constants in this calculation (luminescence counts per second at each time point divided by total remaining counts), the estimated concentration of free Ca 2+ is thus not dependent on absolute cell density [55] . Briefly, 50 μl of each strain was incubated in 500 μl buffer AK S (25 mM HEPES, 125 mM NaCl, 3 mM KCl, 1 mM MgCl 2 and 800 mM Mannitol pH 7.5) and the luminescence counts were recorded. After 60 s, 500 μl of buffer AK S supplemented with 2 mM Ca 2+ was added (to give a final extracellular Ca 2+ concentration of 1 mM) and the counts were recorded for a further 2 min. Then both strains were challenged with a hypoosmotic shock of ~350 mOsm using the addition of 500 μl of double distilled water supplemented with 1 mM Ca 2+ . How to cite this article: Cox, C. D. et al. Selectivity mechanism of the mechanosensitive channel MscS revealed by probing channel subconducting states. Nat. Commun. 4:2137 doi: 10.1038/ncomms3137 (2013).